Recombinant SINEs are formed at high frequency during induced retrotranspositionin vivo Non-long terminal repeat Retrotransposons are referred to as long interspersed nuclear elements (LINEs) and their non-autonomous partners are short interspersed nuclear elements (SINEs). It is believed that an active SINE copy, upon retrotransposition, generates near identical copies of itself, which subsequently accumulate mutations resulting in sequence polymorphism. Here we show that when a retrotransposition-competent cell line of the parasitic protist Entamoeba histolytica , transfected with a marked SINE copy, is induced to retrotranspose, >20% of the newly retrotransposed copies are neither identical to the marked SINE nor to the mobilized resident SINEs. Rather they are recombinants of resident SINEs and the marked SINE. They are a consequence of retrotransposition and not DNA recombination, as they are absent in cells not expressing the retrotransposition functions. This high-frequency recombination provides a new explanation for the existence of mosaic SINEs, which may impact on genetic analysis of SINE lineages, and measurement of phylogenetic distances. Retrotransposons of the non-long terminal repeat (non-LTR) category are generally referred to as long interspersed nuclear elements (LINEs) and their non-autonomous partners are called short interspersed nuclear elements (SINEs) [1] . SINEs are extremely efficient genome invaders. The most well-known SINE, the human Alu element is found in 1.1 million copies in the human genome [2] . Individual SINE copies typically show extensive sequence polymorphism [3] , [4] , [5] . How this polymorphism is generated is not clear, and direct sequence comparison of newly retrotransposed SINE copies with their 'source' copy has not been reported. It should be possible to address this issue using retrotransposition-competent cell lines. In vivo retrotransposition of the human LINE, L1 [6] in cultured cells, and SINEs, Alu [7] and SVA [8] , [9] ; and a LINE/SINE pair from eel [10] , have been well documented. However, analysis of sequence changes in retrotransposed copies compared with the marked SINE copy after a round of retrotransposition has been limited. We have been studying the LINE and SINE elements in the early branching parasitic protist Entamoeba histolytica . These retrotransposons comprise ~11% of the 23-Mb genome [11] , [12] , [13] . EhLINEs belong to the R2 group of non-LTR retrotransposons [14] , [15] , [16] . EhLINEs/SINEs are generally located in intergenic regions [11] , [13] , but not within genes. The 4.8-kb EhLINE1 contains two open reading frames (ORFs) ( Fig. 1a ). ORF2 encodes the reverse transcriptase (RT) and endonuclease (EN) activities typically required for non-LTR element retrotransposition [6] , [17] , [18] , [19] . EhSINE1 (550 bp) is the likely non-autonomous partner of EhLINE1. The two share a 78-bp stretch of sequence homology at their 3′ ends ( Fig. 1a ) [10] , [11] , [20] . Of the 742 EhLINE1 copies in the E. histolytica genome, 88 are full-length, but they lack complete ORFs [13] . Therefore to study retrotransposition in these cells it is necessary to generate a cell line that expresses both ORFs of EhLINE1. Here we report the construction of such a cell line, which expresses ORF2 in a tetracycline (tet)-inducible manner, and can retrotranspose a SINE copy in the presence of tet. This is the first report of active retrotransposition in a parasitic protist cell line. Using this system, we demonstrate a novel feature of high-frequency recombination between SINE copies during retrotransposition. 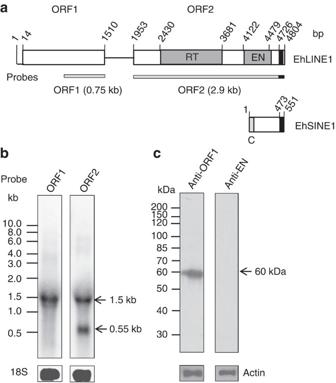Figure 1: Expression of EhLINE1 and EhSINE1 in normally proliferatingE. histolytica. (a) Organization of EhLINE1 and EhSINE111. The ORF2 contains RT and EN domains15. The sequence similarity of 78 bp between EhLINE1 and EhSINE1 at their 3′ ends is shown by a solid black bar. The region marked 'C' (100 bp) in EhSINE1 is conserved in all EhSINEs and may contain the SINE promoter12. (b) Northern hybridization was performed with total cellular RNA isolated from normally proliferating trophozoites with the hybridization probes as indicated in (a). The 0.55-kb band corresponds to EhSINE1 and is seen with ORF2 probe containing the 78-bp common 3′-end. No full-length EhLINE1 transcripts of 4.8 kb are seen. Instead the ORF1 and 2 probes hybridize with a 1.5-kb band, which probably corresponds to transcripts from the abundant truncated EhLINE copies11. (c) Western blotting followed by immunodetection with affinity-purified anti-ORF1 and anti-EN antibodies was performed using total cellular lysate. Band of 60 kDa (ORF1p) is indicated. Anti-actin antibody was used for loading control. Figure 1: Expression of EhLINE1 and EhSINE1 in normally proliferating E. histolytica . ( a ) Organization of EhLINE1 and EhSINE1 [11] . The ORF2 contains RT and EN domains [15] . The sequence similarity of 78 bp between EhLINE1 and EhSINE1 at their 3′ ends is shown by a solid black bar. The region marked 'C' (100 bp) in EhSINE1 is conserved in all EhSINEs and may contain the SINE promoter [12] . ( b ) Northern hybridization was performed with total cellular RNA isolated from normally proliferating trophozoites with the hybridization probes as indicated in ( a ). The 0.55-kb band corresponds to EhSINE1 and is seen with ORF2 probe containing the 78-bp common 3′-end. No full-length EhLINE1 transcripts of 4.8 kb are seen. Instead the ORF1 and 2 probes hybridize with a 1.5-kb band, which probably corresponds to transcripts from the abundant truncated EhLINE copies [11] . ( c ) Western blotting followed by immunodetection with affinity-purified anti-ORF1 and anti-EN antibodies was performed using total cellular lysate. Band of 60 kDa (ORF1p) is indicated. Anti-actin antibody was used for loading control. Full size image A retrotransposition-competent E. histolytica cell-line Although EhSINE1 transcripts are abundantly present in E. histolytica cells [21] , [22] , full-length transcripts of EhLINE1 are not detected ( Fig. 1b ). We show that E. histolytica cells maintained in the lab express ORF1p ( Fig. 1c ), but fail to express detectable levels of ORF2p; hence these cells are not expected to be retrotransposition competent. The study of active retrotransposition requires the construction of a cell line expressing the LINE-encoded ORFs, as achieved with human L1 [6] , which could also retrotranspose SINEs, such as Alu [7] and SVA [8] , [9] . To express the functions required for retrotransposition, we reconstructed the complete ORF2 (lacking any stop codons) by overlapping PCR ( Fig. 2a ), cloned it in a tet-inducible expression vector ( Fig. 2b ) and introduced it into E. histolytica cells to obtain the cell line Eh-ORF2. Our strategy to measure retrotransposition was to introduce in this cell line a plasmid containing a marked EhSINE1 copy (with a 25-bp GC-rich tag), and a known target site of EhSINE1 insertion [15] ( Fig. 2c ). The sequence used as the target site for insertion was identified in a previous study in which we had looked for 'empty' sites in the genome, where a SINE element was missing in one chromosomal copy, but had inserted in another copy of the E. histolytica polyploid genome. The empty versus occupied site was differentiated by PCR amplification with flanking primers. The target site used in this assay was one such sequence with an empty site [15] . Hence, it is a sequence used by the E. histolytica retrotransposition machinery for SINE insertion in vivo . 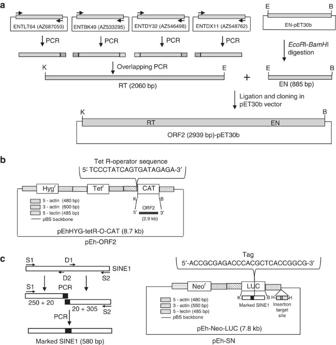Figure 2: Construction of complete ORF2 and pEh-ORF2 and pEh-SN plasmids. (a) Overlapping GSS clones having maximum similarity with consensus sequence of ORF2 of EhLINE1 and lacking any stop codons were selected for reconstruction of ORF2. PCR-amplified fragments of the indicated GSS clones were used in an overlapping PCR to obtain 2,060 bp fragment containing the RT domain, which was later stitched with previously cloned fragment containing the EN domain15to obtain DNA sequence of the full-length ORF2. It was cloned in pET30b vector atKpnI-BamHI sites. Accession numbers of GSS clones are given in brackets K-KpnI, B-BamHI, E-EcoRI. (b) Cloning of ORF2 in place of CAT in the tet-inducible vector pEhHYG-tetR-O-CAT atKpnI andBamHI sites to get pEh-ORF2. The 5′- and 3′-actin and 5′-lectin sequences contain regulatory sequences from theE. histolyticagenes to drive transcription. A sequence of 19 bp inserted between TATA box and ATTCA initiator element in lectin promoter, which acts as a TetR-operator is shown30. (c) Cloning of marked EhSINE1 and insertion target site inE. histolyticavector pEh-Neo-LUC. A 25-bp GC-rich DNA tag (with no match withE. histolyticagenome) was inserted at position 250 from 5′-end in EhSINE1 (555 bp). To insert this tag, the EhSINE1 was first PCR amplified in two fragments, that is, 270 and 325 bp with primer pairs S1-D2 and D1-S2, respectively. The primers D2 and D1 contained an overhang of 20 nucleotides each at their 5′-end corresponding to the tag sequence and had 15 nucleotides complementary to each other. These two fragments were used as templates in a second PCR with primers S1–S2 to yield the 580-bp marked EhSINE1 with 25 bp GC-rich tag. This was cloned inKpnI andBamHI restriction sites by replacing the 1.65-kb LUC. A genomic target site for EhSINE insertion was also provided by inserting the 176-bp DNA fragment containing this site, downstream to 3′-actin sequence at theHindIII (H) site. This site corresponds to the endonuclease nicking hot spot #3 in this fragment, which has been previously described15. It is located 76 nucleotides from 5′-end of this fragment. Figure 2: Construction of complete ORF2 and pEh-ORF2 and pEh-SN plasmids. ( a ) Overlapping GSS clones having maximum similarity with consensus sequence of ORF2 of EhLINE1 and lacking any stop codons were selected for reconstruction of ORF2. PCR-amplified fragments of the indicated GSS clones were used in an overlapping PCR to obtain 2,060 bp fragment containing the RT domain, which was later stitched with previously cloned fragment containing the EN domain [15] to obtain DNA sequence of the full-length ORF2. It was cloned in pET30b vector at Kpn I- BamH I sites. Accession numbers of GSS clones are given in brackets K- Kpn I, B- BamH I, E- EcoR I. ( b ) Cloning of ORF2 in place of CAT in the tet-inducible vector pEhHYG-tetR-O-CAT at Kpn I and BamH I sites to get pEh-ORF2. The 5′- and 3′-actin and 5′-lectin sequences contain regulatory sequences from the E. histolytica genes to drive transcription. A sequence of 19 bp inserted between TATA box and ATTCA initiator element in lectin promoter, which acts as a TetR-operator is shown [30] . ( c ) Cloning of marked EhSINE1 and insertion target site in E. histolytica vector pEh-Neo-LUC. A 25-bp GC-rich DNA tag (with no match with E. histolytica genome) was inserted at position 250 from 5′-end in EhSINE1 (555 bp). To insert this tag, the EhSINE1 was first PCR amplified in two fragments, that is, 270 and 325 bp with primer pairs S1-D2 and D1-S2, respectively. The primers D2 and D1 contained an overhang of 20 nucleotides each at their 5′-end corresponding to the tag sequence and had 15 nucleotides complementary to each other. These two fragments were used as templates in a second PCR with primers S1–S2 to yield the 580-bp marked EhSINE1 with 25 bp GC-rich tag. This was cloned in Kpn I and BamH I restriction sites by replacing the 1.65-kb LUC. A genomic target site for EhSINE insertion was also provided by inserting the 176-bp DNA fragment containing this site, downstream to 3′-actin sequence at the Hind III (H) site. This site corresponds to the endonuclease nicking hot spot #3 in this fragment, which has been previously described [15] . It is located 76 nucleotides from 5′-end of this fragment. Full size image Retrotransposition events occurring at this target site were scored without using selection pressure. Being PCR-based, we expect the scoring to be very sensitive. The doubly transfected cell line (Eh-ORF2-SN) expressed 2.9 kb ORF2 transcript ( Fig. 3a ) and ORF2p (111 kDa) ( Fig. 3b ) in a tet-inducible manner. 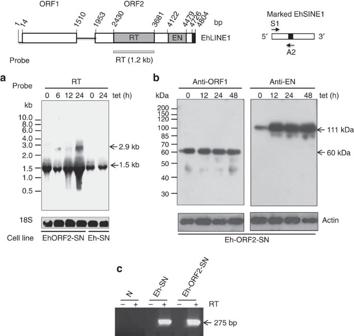Figure 3: Expression analysis of EhLINE1 and EhSINE1 in the Eh-ORF2-SN cell line. (a) Northern hybridization was performed with total cellular RNA isolated from cells doubly transfected with pEh-ORF2 and pEh-SN (Eh-ORF2-SN), or with pEh-SN and EhHYG-tetR-O-CAT vector (Eh-SN). Position of the hybridization probe in EhLINE1 is indicated in upper panel. The 2.9-kb band corresponds to the ORF2 transcript after induction with 10 μg ml−1tet. No full-length EhLINE1 transcripts of 4.8 kb are seen. (b) Western blotting followed by immunodetection with affinity-purified anti-ORF1 and anti-EN antibodies was performed using total cellular lysate from the Eh-ORF2-SN cell line. Bands of 60 kDa (ORF1p) and 111 kDa (ORF2p) are indicated. Anti-actin antibody was used for loading control. (c) The marked EhSINE1 transcript was detected by RT–PCR with total RNA. RT reaction was with primer A2 from the tag followed by PCR with primers S1 and A2 (position of primers shown in upper panel). The expected size PCR product (275 bp) was obtained. No amplicon was obtained from untransfected cells (N). The constitutive expression of ORF1p (60 kDa) was unaltered on tet induction ( Fig 3b ). This cell line also expressed the transcript corresponding to the marked SINE1 ( Fig 3c ). In the presence of tet, this cell line is expected to be retrotransposition competent. We added tet to cultures in early log phase and harvested the cells after 48 h (late log). We scored retrotransposition of the marked SINE copy to the insertion target site by PCR amplification of total genomic DNA using two sets of primer pairs to discount the possibility of PCR artefacts ( Fig. 4 ). The identity of the amplicons was further confirmed by Southern hybridization with the marked SINE probe. We did not obtain amplicons in the absence of tet, whereas in the presence of tet, specific amplicons expected from the mobilization of the marked SINE to the insertion site were obtained with both primer pairs ( Fig. 4a,b ). We also did not obtain amplicons when tet was added to a cell line containing the marked SINE and insertion hotspot but lacking ORF2 (Eh-SN). A hallmark of retrotransposition is the generation of target site duplications (TSD). We induced retrotransposition by tet addition in three independently grown cultures and sequenced the flanking sequences of thirteen random clones of the amplicons. We predominantly found a 22-bp TSD ( Fig. 4c ), which matched exactly in size and sequence with the TSD found at this insertion hotspot at its genomic location [15] . We did not find insertion at any region in the 176-bp fragment other than the hotspot. Therefore, based on three criteria namely, strict requirement of ORF2p expression for mobilization, specific insertion into the retrotransposition hotspot and the 22-bp TSDs accompanying the insertion, we conclude that the events scored by us are due to retrotransposition and not due to DNA recombination. This is the first demonstration of active retrotransposition in a primitive protist. Figure 3: Expression analysis of EhLINE1 and EhSINE1 in the Eh-ORF2-SN cell line. ( a ) Northern hybridization was performed with total cellular RNA isolated from cells doubly transfected with pEh-ORF2 and pEh-SN (Eh-ORF2-SN), or with pEh-SN and EhHYG-tetR-O-CAT vector (Eh-SN). Position of the hybridization probe in EhLINE1 is indicated in upper panel. The 2.9-kb band corresponds to the ORF2 transcript after induction with 10 μg ml −1 tet. No full-length EhLINE1 transcripts of 4.8 kb are seen. ( b ) Western blotting followed by immunodetection with affinity-purified anti-ORF1 and anti-EN antibodies was performed using total cellular lysate from the Eh-ORF2-SN cell line. Bands of 60 kDa (ORF1p) and 111 kDa (ORF2p) are indicated. Anti-actin antibody was used for loading control. ( c ) The marked EhSINE1 transcript was detected by RT–PCR with total RNA. RT reaction was with primer A2 from the tag followed by PCR with primers S1 and A2 (position of primers shown in upper panel). The expected size PCR product (275 bp) was obtained. No amplicon was obtained from untransfected cells (N). 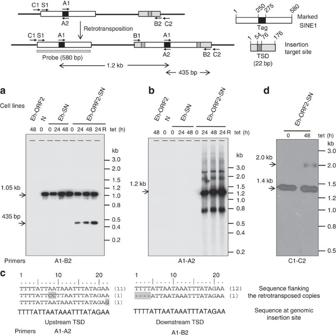Figure 4: Tet-induced retrotransposition of the marked EhSINE1 at the target site. The top panel shows the construct containing the marked EhSINE1 (580 bp, hollow rectangle) with a 25-bp GC-rich tag (black rectangle) cloned in the vector pEh-Neo-LUC. The 176-bp fragment (grey box) containing an insertion target site (dark grey box) is shown. Genomic DNA was isolated from untransfected cells (N), single transfectant (Eh-ORF2) and double transfectants (Eh-ORF2-SN and Eh-SN) induced with tet for indicated times. PCR was carried out with the indicated primers whose location is shown in the top panel. PCR products were detected by using double-stranded probe from the marked SINE1. 24R refers to EhORF2-SN cells induced with tet for 24 h and further grown for 24 h in the absence of tet. Results of Southern hybridization are shown in panelsa,bandd. Panelcshows sequence alignment of upstream and downstream TSDs in 13 retrotransposed copies, obtained by PCR amplification with primers (A1–A2 and A1–B2). The number of copies with the 22-bp TSD identical to the TSD observed at the genomic insertion at the same site is given in brackets. The mismatches are shaded in grey. All retrotransposition events occurred only at indicated target site and nowhere else in the 176-bp fragment. Full size image Figure 4: Tet-induced retrotransposition of the marked EhSINE1 at the target site. The top panel shows the construct containing the marked EhSINE1 (580 bp, hollow rectangle) with a 25-bp GC-rich tag (black rectangle) cloned in the vector pEh-Neo-LUC. The 176-bp fragment (grey box) containing an insertion target site (dark grey box) is shown. Genomic DNA was isolated from untransfected cells (N), single transfectant (Eh-ORF2) and double transfectants (Eh-ORF2-SN and Eh-SN) induced with tet for indicated times. PCR was carried out with the indicated primers whose location is shown in the top panel. PCR products were detected by using double-stranded probe from the marked SINE1. 24R refers to EhORF2-SN cells induced with tet for 24 h and further grown for 24 h in the absence of tet. Results of Southern hybridization are shown in panels a , b and d . Panel c shows sequence alignment of upstream and downstream TSDs in 13 retrotransposed copies, obtained by PCR amplification with primers (A1–A2 and A1–B2). The number of copies with the 22-bp TSD identical to the TSD observed at the genomic insertion at the same site is given in brackets. The mismatches are shaded in grey. All retrotransposition events occurred only at indicated target site and nowhere else in the 176-bp fragment. Full size image Analysis of the newly retrotransposed copies of EhSINEs Next we checked the sequences of the newly retrotransposed copies. To recover all retrotransposition events due to SINEs, we obtained amplicons using the primer pair C1/C2 ( Fig. 4d ), which gave a 1.4 kb amplicon from the parent plasmid and a 2.0 kb amplicon expected from events where a SINE copy had retrotransposed at the insertion hotspot. We did not obtain bands shorter than 2.0 kb, which shows that in our system the predominant retrotransposition events are contributed by full-length SINEs. This is expected, as truncated SINE transcripts are not seen, whereas full-length transcripts are abundant in E. histolytica [23] , [24] . This also shows that 5′-truncations are not common during EhSINE retrotransposition. We cut out the 2.0-kb band and reamplified it using the primer pair B1/B2 ( Fig. 4 ). We cloned the 0.8-kb amplicon so obtained, and sequenced 23 randomly selected clones. The data showed that the sequences belonged to three different categories ( Table 1 ) namely; Set I, a set of ten sequences matching completely with the marked SINE; Set II, a set of eight sequences lacking the tag and matching with genomic SINE copies; and Set III, a set of five sequences containing the 25-bp tag at the expected location but, otherwise, matching with genomic SINEs rather than the marked SINE. In these five instances of set III, the tag had associated itself with genomic SINE sequences. Characteristics of each set are as follows. Of the ten sequences in set I, seven were 100% identical to the marked SINE, and three had one mismatch each. The nucleotide position of the mismatch is indicated in Table 1, and shows that the mismatches are not clustered. In set II, all eight sequences lacked the tag and showed only 95–96% sequence identity (19–27 mismatches) with the marked SINE. As this level of identity is seen between random genomic EhSINE1 copies, these sequences would not have arisen from the marked SINE. Rather they may correspond to genomic SINEs. It is estimated that 142 SINE copies are transcribed in E. histolytica [12] , some of which may be mobilized in our cell line upon tet induction.Sequence comparison showed that seven of the eight sequences in set II indeed showed 98–99% identity with genomic EhSINE1 sequences found in the E. histolytica EST database (3–11 mismatches with best data base hits when compared with the full-length SINE sequence; Table 1 , set II). The number of mismatches seen in separate comparisons of 5′-half and 3′-half with the EhSINE1 sequences in the data base is explained later. We confirmed that the database comparison was valid, as random check of PCR amplicons from four of these loci from our cultured cells showed 100% sequence match with the database. These events therefore resulted from the mobilization of transcribed genomic SINE copies and not from the marked SINE copy. Table 1 Sequence analysis of newly retrotransposed SINE copies. Full size table In set III, all five sequences had the 25-bp tag but, surprisingly, showed only 94–95% overall sequence identity (22–27 mismatches) with the marked SINE. When we searched these sequences (minus the tag) for identical hits in the E. histolytica data base we found at best 94–98% matches (11–28 mismatches in the full length SINE sequence). However, when we searched the sequence on either side of the tag separately (5′-half and 3′-half of each SINE separately; Table 1 , set III), 98–100% matches were obtained, and each side matched with different genomic SINE sequences (accession codes are provided in Supplementary Table S1 ). Thus it seems that these five sequences are recombinants, derived from at least three different SINE sequences, one of them being the marked SINE and two belonging to different genomic SINEs. If the tag was acquired by the genomic SINE copies through a DNA-recombination event before retrotransposition, the tag should be present in the transcripts of these SINEs. To check this, we took total RNA from Eh-ORF2-SN cells induced with tet and did RT–PCR in two parts using primers from the tag and from SINE sequences at either end ( Fig. 5a,b ). We sequenced ten random clones of the amplicons from each side. All clones were identical only to the marked SINE sequence, showing that tag-containing transcripts arose only from the marked SINE copy. To further check if the recombinants existed before the induction of retrotransposition, we performed genomic PCR with DNA from Eh-ORF2-SN cells before tet addition using primers from the tag and opposite primers specific to the five mobilized copies of set III ( Fig. 5c ). No amplicons were obtained with this DNA, whereas DNA from cells after tet addition gave the expected amplicons, showing that the tag was not associated with these sequences before retrotransposition. 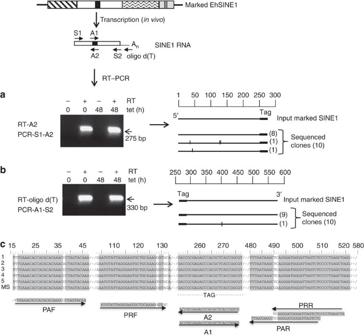Figure 5: Sequence changes in SINEs were not due to transcription or genomic recombination. Total cellular RNA was isolated from the Eh-ORF2-SN cells grown for 48 h with 10 μg ml−1tet and cDNA was synthesized with MuMLV-RT by using primers shown in the upper panel. Primers S1 and S2 are from conserved SINE sequences and would amplify genomic as well as marked SINE1. (a) RT reaction with primer A2 followed by PCR with primers S1-A2. The amplicon of 275 bp thus obtained was cloned in pGEMTEasy vector and ten random clones were selected for sequencing. The DNA sequence of SINE1 in these clones is represented by bold lines with eight clones having sequence identical to input-tagged EhSINE1 and two clones having three and one mismatches, respectively (represented by vertical lines). (b) Same as in (a), with indicated RT–PCR primers to obtain the SINE sequence 3′ of the tag. As EhSINEs are polyadenylated at 3′ ends21,22, RT reaction was primed with oligo d(T). (c) Multiple alignment of the five clones of set III and the marked EhSINE1 (MS) shows the location of primers for genomic PCR. Primer pairs PRF-A2 and A1-PRR were used with total genomic DNA to check if tag-containing set III sequences already existed in the genome before induction of retrotransposition with tet. Primer pair PAF-PAR was derived from conserved sequences and served as positive control. Figure 5: Sequence changes in SINEs were not due to transcription or genomic recombination. Total cellular RNA was isolated from the Eh-ORF2-SN cells grown for 48 h with 10 μg ml −1 tet and cDNA was synthesized with MuMLV-RT by using primers shown in the upper panel. Primers S1 and S2 are from conserved SINE sequences and would amplify genomic as well as marked SINE1. ( a ) RT reaction with primer A2 followed by PCR with primers S1-A2. The amplicon of 275 bp thus obtained was cloned in pGEMTEasy vector and ten random clones were selected for sequencing. The DNA sequence of SINE1 in these clones is represented by bold lines with eight clones having sequence identical to input-tagged EhSINE1 and two clones having three and one mismatches, respectively (represented by vertical lines). ( b ) Same as in ( a ), with indicated RT–PCR primers to obtain the SINE sequence 3′ of the tag. As EhSINEs are polyadenylated at 3′ ends [21] , [22] , RT reaction was primed with oligo d(T). ( c ) Multiple alignment of the five clones of set III and the marked EhSINE1 (MS) shows the location of primers for genomic PCR. Primer pairs PRF-A2 and A1-PRR were used with total genomic DNA to check if tag-containing set III sequences already existed in the genome before induction of retrotransposition with tet. Primer pair PAF-PAR was derived from conserved sequences and served as positive control. Full size image We conclude that recombinant SINEs are formed consequent to retrotransposition. The process is rapid, as we scored these events within 48 h of retrotransposition induction, and occurs at high frequency (>20% of total events scored). Some of the events in set II might also be recombinants, as the number of mismatches reduced when the 5′ and 3′ halves of each sequence were searched separately with the database ( Table 1 ). Although the number of mismatches in a full-length comparison ranged from 3 to 20, this number became 0 to 4 when matches were searched only for the 5′-half, and was 0 to 5 when matches were searched for the 3′-half. In two cases the sequence had to be matched in three parts (5′, 3′, and middle) to get minimum mismatches. Retrotransposition-competent cell lines have greatly assisted in understanding the mechanism of non-LTR retrotransposition in vivo [6] , [7] , [8] , [9] , [10] . Here we report the first such system in a parasitic protist E. histolytica . Our results show that in this organism the newly retrotransposed EhSINE copies undergo high-frequency recombination, not known earlier to take place in this class of non-LTR retrotransposons. Chimeric molecules arising from reverse transcripts have been observed in yeast Ty elements, and were attributed to gene conversion [23] , whereas in retroviruses high-frequency recombination occurs during reverse transcription of the two co-packaged RNAs in the virion as a result of template switching [24] . In non-LTR elements, tripartite chimeric LINEs have earlier been reported in a fungal genome [25] , and in mammalian genomes U6/L1 pseudogene chimeras have been experimentally demonstrated [26] . However, recombination between multiple copies of the same SINE family during retrotransposition is a novel observation. The demonstrated properties of RT to displace the RNA template during complementary DNA (cDNA) synthesis, and to perform multiple template jumping [27] , [28] could lead to these recombinants. The template jumping activity reported for non-LTR retrotransposons involves end-to-end jumping between the template RNAs, and this is frequently accompanied by the addition of non-templated nucleotides at the junction. The recombinant SINEs reported here are not generated by end-to-end jumping. They would require the RT to switch at internal positions from one template RNA to the next. Such switching has not been reported for the RT encoded by non-LTR elements and needs to be explored further. Our data ( Table 1 ) suggests that, more frequently, no switches take place during retrotransposition (at least 10 out of 23 occurrences; set I); but multiple switching events are commonly encountered. In set II, four events (sequences 2, 3, 4 and 8) probably did not involve any switch, whereas two (numbers 1 and 7) could involve one switch each, and the remaining two (numbers 5 and 6) could involve two switches each. In set III, all five events seemed to be a result of two switches. This may be due to the small sample size in this set. If such recombination is indeed common, one should expect the E. histolytica SINE population to display a prominent mosaic structure. To check this, we did multiple alignment of 63 full-length EhSINE1 copies thought to have retrotransposed most recently [12] , and looked at all positions that were polymorphic in at least 20% of the SINEs. We found 16 such positions. We organized the sequences in these positions in blocks of four, and clustered the positions with identical sequences into sets in the leftmost block ( Fig. 6 ). Upon aligning these sequences with the next block of four, it is evident that the sequences of identical sets in the first block segregate out and associate in various combinations. Nine sets in the first block associated with twelve sets in the second block in 34 different combinations. The combination of patterns in all four blocks taken together showed clear indication of mosaic formations that would be expected to arise from internal template jumps during retrotransposition. 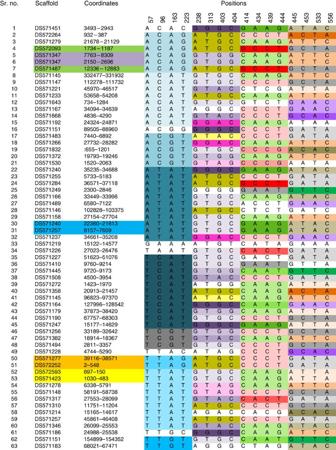Figure 6: Polymorphic sites in the EhSINE1 population are distributed in a mosaic pattern. The coordinates of the 63 full-length EhSINE1 copies selected for analysis are shown on the left. These copies were selected because they are thought to have retrotransposed most recently12. Sequences of the 63 copies were aligned and nucleotide positions varying in at least 12 copies were selected. In all, 16 such positions found are displayed. Blocks of four consecutive positions with the same sequence have been given the same colour for clarity. The five identical pairs found are indicated by same shading in the left column. Figure 6: Polymorphic sites in the EhSINE1 population are distributed in a mosaic pattern. The coordinates of the 63 full-length EhSINE1 copies selected for analysis are shown on the left. These copies were selected because they are thought to have retrotransposed most recently [12] . Sequences of the 63 copies were aligned and nucleotide positions varying in at least 12 copies were selected. In all, 16 such positions found are displayed. Blocks of four consecutive positions with the same sequence have been given the same colour for clarity. The five identical pairs found are indicated by same shading in the left column. Full size image Although sequence analysis of human Alu subfamilies showed the existence of mosaic elements [29] these were not experimentally found [7] , [8] , [9] . Mosaics could have been missed in these studies because of the smaller number of retrotransposition events scored, and the selection pressure used. Our results are the first direct demonstration that SINE copies engage in active sequence exchange during retrotransposition, leading to the rapid spread of the sequence tag to the SINE population, and generation of diversity. As mRNA transcripts are also templates of the same retrotransposition machinery during retropseudogene formation, it will be interesting to see if mRNA transcripts could also engage in similar recombination during reverse transcription [29] . Cell culture and growth conditions Trophozoites of E. histolytica strain HM-1:IMSS (clone 6) were axenically maintained and stable transfectants were obtained as described previously [30] . Single and double transfectants were maintained with 10 μg ml −1 of Hygromycin B or G418 or both. Immunodetection Western analysis was performed with 100 μg of total cell lysates separated on 10% SDS–polyacrylamide gel electrophoresis and blotted using Mini-Trans Blot Electrophoretic Cell (Bio-Rad). Polyclonal antibodies, anti-EN (mouse) and anti-ORF1 (rabbit) were raised against each his-tagged recombinant protein purified through Ni-NTA agarose. 1:5,000 dilution of each anti-serum followed by HRP-conjugated secondary antibodies (1:10,000, Sigma) were used to detect respective polypeptides. ECL reagents were used for visualization (Millipore). DNA sequence analysis The genome sequence of E . histolytica having 1529 scaffolds was downloaded from NCBI database, with accession IDs AAFB00000000 , and was searched (using BLAST tool) for matches with the sequences of retrotransposed copies of Sets II and III ( Table 1 and Supplementary Table S1 ). In all, 25 nucleotides from both the ends of these copies were removed before BLAST analysis to remove any bias due to other factors (for example, addition of non-templated nucleotides during the RT reaction). Hits showing 100% coverage and maximum similarity were recorded. The coordinates of EhSINEs in various scaffolds are as per previous report [12] . How to cite this article: Yadav, V. P. et al . Recombinant SINEs are formed at high frequency during induced retrotransposition in vivo . Nat. Commun. 3:854 doi: 10.1038/ncomms1855 (2012).